A shift of the TOR adaptor from Rictor towards Raptor by semaphorin inC. elegans The target of rapamycin (TOR), a central regulator for cell growth and metabolism, resides in the two functionally distinct complexes TORC1 and TORC2, which are defined by their adaptors Raptor and Rictor, respectively. How the formation of the two TORCs is orchestrated remains unclear. Here we show the control of TOR partnering by semaphorin-plexin signalling in Caenorhabditis elegans . In semaphorin and plexin mutants, TOR-Raptor association decreases whereas TOR-Rictor association increases, concomitantly with TORC1 down- and TORC2 up-regulation. Epidermal defects in the mutants are suppressed by inhibiting TORC2 or reinforcing TORC1 signalling. Conversely, inhibition of TORC1 signalling phenocopies the mutants. Thus, our results indicate that TORC formation is a singularly important step in semaphorin signalling that culminates in diverse outcomes including TORC1-promoted messenger RNA translation and TORC2-regulated cytoskeletal remodelling. Signals of semaphorins, through their predominant receptors plexins, regulate a wide range of morphogenetic events [1] . Key regulators mediating the signals include cytoskeleton-relevant Rho family GTPases and their effectors such as actin-depolymerizing factor/cofilin [2] , [3] . Importantly, messenger RNA translation, whose rates are defined by phosphorylation states of translation factors eIF2α and 4EBP [4] , is augmented by semaphorins. In vertebrate cultured neurons, semaphorin-induced growth cone responses require rapid mRNA translation through the 4EBP–eIF4F pathway [5] , [6] . Recently, our genetic work utilizing the system of 'ray' morphogenesis in Caenorhabditis elegans showed that stimulated translation, which involves phosphorylation control of eIF2α, mediates the semaphorin signal [7] . mRNA species that are translated in response to semaphorins include cofilin and RhoA [6] , [7] , [8] , suggesting that activation of cytoskeletal regulators, as well as their de novo synthesis, are essential for semaphorin signalling. Mechanisms of the signalling, however, have not been fully elucidated. The target of rapamycin (TOR), an evolutionarily conserved serine/threonine kinase, is a pivotal regulator for cell growth, morphogenesis and proliferation, which governs and integrates signals from a variety of environmental stimuli [9] , [10] . TOR resides as a catalytic subunit in two biochemically and functionally distinct multiprotein complexes referred to as TOR complex 1 (TORC1) and TOR complex 2 (TORC2), which are defined by the TOR-associated adaptor proteins Raptor (regulatory associated protein of mTOR) and Rictor (rapamycin-insensitive companion of TOR), respectively [11] , [12] , [13] , [14] . An upstream activator of TORC1 is Rheb GTPase [15] , the activity of which can be switched off by the GTPase-activating protein complex TSC1/TSC2 (refs 16 , 17 , 18 ). Signalling through TORC1 culminates in the promotion of mRNA translation by phosphorylating translational regulators 4EBP and S6K [19] . Functions of TORC2 are less well defined than those of TORC1, but recent work has indicated that TORC2 is involved in remodelling of actin architecture through PKCα and Rac GTPase [13] , [14] , [20] . In addition, TORC2 contributes to maintaining cellular viability and size by phosphorylating AKT/protein kinase B [21] , [22] , [23] . Rictor is required for TORC2 integrity and substrate specificity, though very little is known about the regulation of TORC2. Another elusive issue is whether and how the two TORCs integrities are orchestrated in vivo . In this study, we report a new link between the semaphorin input and TOR partnering. Through genetic analyses in C. elegans , we demonstrate that semaphorin activates TORC1 and simultaneously inhibits TORC2 by promoting a shift of the TOR adaptor from Rictor towards Raptor. Furthermore, not only activation of TORC1 but inhibition of TORC2 is also required for semaphorin-induced epidermal cellular morphogenesis. Together, we propose that TOR integrates and transduces the upstream semaphorin signal by acting as a central commander that orchestrates multiple downstream cascades. Loss of Rictor suppresses the defects in semaphorin mutants In C. elegans , signalling of membrane-bound semaphorins (SMP-1 & SMP-2; SMP) through plexin (PLX-1) regulates the arrangement of rays: bilateral nine-paired sensilla found in a male tail [24] , [25] . Each protruding ray consists of three cells including a support cell and two neuronal cells, all of which originate from an epidermal cellular cluster [26] . At the early third larval stage (L3 stage), several rounds of epidermal cell divisions in a tail generate nine sets of clusters as well as extra hypodermal Rn.p cells ( n =1–9). One major role of the SMP–PLX-1 signal is to posteriorly shift the boundary between R1.p and R2.p at the late L3 stage [24] . Because the ray 1-differentiating cluster (cluster 1) is destined to be located at the R1.p–R2.p boundary [27] , its posterior shift allows for the location of cluster 1 adjacent to cluster 2. This is how, in wild-type adults, ray 1 is juxtaposed to ray 2. By contrast in plx-1 and smp-1 smp-2 mutants, the R1.p–R2.p boundary fails to undergo the posterior shift and thus cluster 1 remains situated anteriorly ( Fig. 1a ), which consequently leads to anterior displacement of ray 1 at the adult stage ( Fig. 1b ). The ray 1 phenotype in plx-1 mutants is markedly rescued by expressing wild-type plx-1 under the promoter of lin-32 gene ( lin-32 p), a ray lineage-specific driver [7] , [28] ( Fig. 1c ). 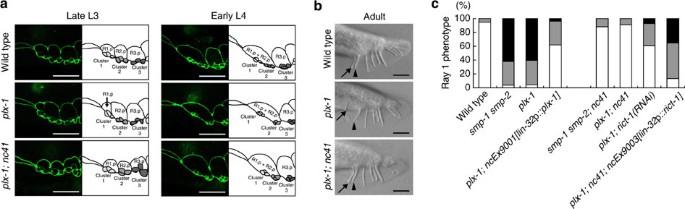Figure 1: Loss ofrict-1function suppresses the ray 1 phenotype inplx-1andsmp-1 smp-2mutants. (a) Configurations of epidermal ray precursor cells visualized withajm-1∷gfpin a wild-type, aplx-1mutant, and aplx-1;rict-1(nc41) mutant animal at the late L3 stage and the early L4 stage. Schematic drawings illustrating the contours of cells are also given. Anterior is left, and dorsal is top. Scale bars, 10 μm. (b) Nomarski images of adult male tails. Ray 1 (arrow), which is located close to ray 2 (arrowhead) in a wild type, is located abnormally at the anterior position in aplx-1mutant, but it is reverted to the normal position in aplx-1;rict-1(nc41) mutant animal. Anterior is left, and dorsal is top. Scale bars, 10 μm. (c) Penetrance of the ray 1 phenotype in adults of the indicated genotypes. For the quantitative evaluation, the ray 1 phenotypes are categorized into either Level 1 (normal), Level 2 (mildly defective), or Level 3 (severely defective), which are represented by white, grey or black segment of each bar, respectively.n=215–234 for each genotype. Figure 1: Loss of rict-1 function suppresses the ray 1 phenotype in plx-1 and smp-1 smp-2 mutants. ( a ) Configurations of epidermal ray precursor cells visualized with ajm-1 ∷ gfp in a wild-type, a plx-1 mutant, and a plx-1 ; rict-1 ( nc41 ) mutant animal at the late L3 stage and the early L4 stage. Schematic drawings illustrating the contours of cells are also given. Anterior is left, and dorsal is top. Scale bars, 10 μm. ( b ) Nomarski images of adult male tails. Ray 1 (arrow), which is located close to ray 2 (arrowhead) in a wild type, is located abnormally at the anterior position in a plx-1 mutant, but it is reverted to the normal position in a plx-1 ; rict-1 ( nc41 ) mutant animal. Anterior is left, and dorsal is top. Scale bars, 10 μm. ( c ) Penetrance of the ray 1 phenotype in adults of the indicated genotypes. For the quantitative evaluation, the ray 1 phenotypes are categorized into either Level 1 (normal), Level 2 (mildly defective), or Level 3 (severely defective), which are represented by white, grey or black segment of each bar, respectively. n =215–234 for each genotype. Full size image To investigate the downstream events of SMP signalling, we conducted a screen for suppressors of plx-1 mutation and isolated a recessive allele, nc41 , which almost fully suppressed the ray phenotype in mutants ( Fig. 1a–c ). No abnormality was found in the ray configuration in nc41 single mutants ( Supplementary Table S1 ). nc41 was mapped to the right arm of linkage group II and was shown through the sequencing to be a 470-bp deletion within rict-1 gene ( Supplementary Fig. S1a and b ), which encodes a protein weakly orthologous to Rictor [29] , [30] . Nucleotides 3,538–3,586 (49 bases) corresponding to part of the 12th exon are deleted in the nc41 -type rict-1 transcript, which produces a nonsense frame-shift leading to the premature opal codon at the predicted 1,200th codon ( Supplementary Fig. S1c ). Knockdown of rict-1 by RNAi suppressed the plx-1 mutant phenotype, whereas wild-type rict-1 expression under the lin-32 p reversed the suppression by nc41 ( Fig. 1c ). Thus, we concluded that nc41 is a loss-of-function rict-1 allele, which is responsible for suppressing the ray 1 phenotype in plx-1 and smp-1 smp-2 mutants. C. elegans Raptor and Rictor define TORC1 and TORC2 In other organisms, Rictor binds TOR to form a multiprotein complex TOR complex 2 (TORC2) [13] , [14] . Independent of TORC2, TOR also forms the complex TORC1 with its defining component Raptor [11] , [12] . To examine TORC formation in C. elegans , we cloned complementary DNAs for TOR ( let-363 ) [31] , Raptor ( daf-15 ) [32] and Rictor ( rict-1 ), and tagged them at their 5′ ends with FLAG , Myc and HA oligonucleotides, respectively. Then, we generated a transgenic line expressing LET-363, DAF-15 and RICT-1 placed under the lin-32 p, together with wild-type plx-1 cDNA placed under a heat-shock promoter ( hs p) ( Fig. 2a ). The resultant line expressing these transgenes seems to be physiologically balanced; no interference with the ray 1 phenotype was observed in the background of wild-type, plx-1 and smp-1 smp-2 mutants ( Supplementary Table S1 ). We also generated a line expressing epitope-tagged LET-363, DAF-15 and RICT-1 under the promoter of unc-54 , a gene specific to body wall muscles, where plx-1 expression does not overlap [24] ( Fig. 2a ). After retrieval of transgenic males at L3–L4 stages, FLAG ∷ LET-363-, Myc ∷ DAF-15- or HA ∷ RICT-1-containing complexes were immunoprecipitated with antibodies against their respective epitope tags and the immunocomplex (IP) was analysed. In both ray precursor cells ( lin-32 -positive) and muscle cells ( unc-54 -positive), the LET-363 IP contained both DAF-15 and RICT-1 ( Fig. 2b ). On the other hand, the DAF-15 IP contained LET-363 but not RICT-1, whereas the RICT-1 IP contained LET-363 but not DAF-15 ( Fig. 2b ). Thus, similar to Raptor and Rictor in other organisms, C. elegans DAF-15 and RICT-1 also define TORC1 and TORC2, respectively. In another line expressing nc41 -type RICT-1 together with LET-363 and DAF-15 under the lin-32 p, LET-363–RICT-1 association was largely abolished ( Fig. 2c ), indicating that TORC2 signalling is blocked by rict-1(nc41) deletion. 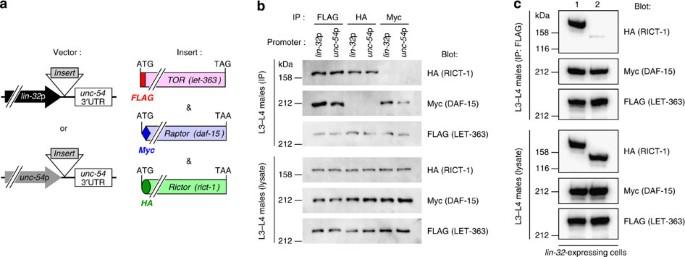Figure 2: DAF-15 and RICT-1 define TORC1 and TORC2, respectively. (a) Schemes of expression constructs for FLAG-tagged TOR (LET-363), Myc-tagged Raptor (DAF-15), and HA-tagged Rictor (RICT-1), all of which are placed under either thelin-32promoter or theunc-54promoter. (b) Mutually exclusive association of DAF-15 and RICT-1 with LET-363. Transgenic L3–L4 males expressing epitope-tagged RICT-1, DAF-15 and LET-363 proteins under thelin-32p (ncEx9005) or theunc-54p (ncEx9007) were lysed, and proteins were immunoprecipitated with antibodies against the indicated tags. The immunocomplex (IP) and lysates were analysed by immunoblotting. (c) Abolished association ofnc41-type RICT-1 with LET-363. Transgenic L3–L4 males expressing wild-type RICT-1 (lane 1:ncEx9005) ornc41-type RICT-1 (lane 2:ncEx9008) together with DAF-15 and LET-363 under thelin-32p were lysed, and FLAG∷LET-363 proteins were immunoprecipitated. The FLAG-precipitated IP and lysates were analysed by immunoblotting. Figure 2: DAF-15 and RICT-1 define TORC1 and TORC2, respectively. ( a ) Schemes of expression constructs for FLAG-tagged TOR (LET-363), Myc-tagged Raptor (DAF-15), and HA-tagged Rictor (RICT-1), all of which are placed under either the lin-32 promoter or the unc-54 promoter. ( b ) Mutually exclusive association of DAF-15 and RICT-1 with LET-363. Transgenic L3–L4 males expressing epitope-tagged RICT-1, DAF-15 and LET-363 proteins under the lin-32 p ( ncEx9005 ) or the unc-54 p ( ncEx9007 ) were lysed, and proteins were immunoprecipitated with antibodies against the indicated tags. The immunocomplex (IP) and lysates were analysed by immunoblotting. ( c ) Abolished association of nc41 -type RICT-1 with LET-363. Transgenic L3–L4 males expressing wild-type RICT-1 (lane 1: ncEx9005 ) or nc41 -type RICT-1 (lane 2: ncEx9008 ) together with DAF-15 and LET-363 under the lin-32 p were lysed, and FLAG ∷ LET-363 proteins were immunoprecipitated. The FLAG-precipitated IP and lysates were analysed by immunoblotting. Full size image Active TORC1 and inactive TORC2 mediate semaphorin signal To address whether perturbed TORC formation by rict-1 mutation is responsible for the suppression of the ray phenotype in plx-1 and smp-1 smp-2 mutants, we knocked-down C. elegans LST8 ( CeLST8 ), whose mammalian orthologue is reportedly essential for signalling of TORC2 but is dispensable for that of TORC1 (ref. 23 ). CeLST8 knockdown markedly suppressed the plx-1 mutant phenotype ( Fig. 3a ). Furthermore, the knockdown obliterated LET-363–RICT-1 association and, to our surprise, increased LET-363–DAF-15 association ( Fig. 3b ). We also found that rict-1 knockdown resulted in an increase in LET-363–DAF-15 association, and daf-15 knockdown, likewise, resulted in an increase in LET-363–RICT-1 association, suggesting a competitive relationship between DAF-15 and RICT-1 for binding to LET-363 ( Supplementary Fig. S2 ). Thus, we presumed that, in addition to decreased TORC2 signalling, increased TORC1 signalling might be involved in bypassing the SMP signal. To examine the possible contribution of increased TORC1 to suppression, we overexpressed DAF-15 under the lin-32 p, and found that the phenotypes in plx-1 and smp-1 smp-2 mutant were partially suppressed ( Fig. 3c ). We also tested whether loss of putative TORC1 inhibitors had a similar suppressive effect on the plx-1 mutant phenotype as DAF-15 overexpression did. LKB1 exists in a heterotrimeric complex with two accessory proteins, Ste20-related adaptor protein (STRAD) and MO25. This complex phosphorylates and activates AMPK, thereby inhibiting the TORC1 pathway [33] . Loss of LKB1 ( par-4 ), STRAD ( strd-1 ), catalytic α subunit of AMPK ( aak-1 & aak-2 ) and β subunit of AMPK ( aakb-1 ) [34] , [35] , [36] partially suppressed the plx-1 mutant phenotype ( Fig. 3d ). These results suggest that, in addition to TORC2 inhibition, TORC1 activation partially contributes to bypassing the SMP signal. 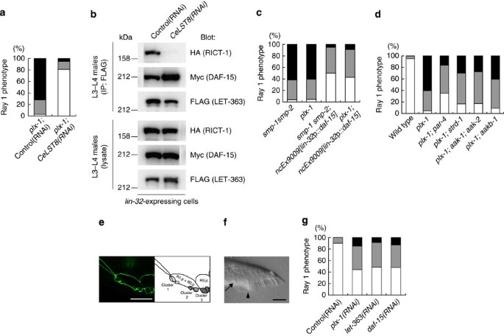Figure 3: TORC2 inhibition and/or TORC1 activation bypass the SMP signal. (a) Quantitative ray 1 phenotype caused byCeLST8knockdown in theplx-1mutant background. (b) Transgenic L3–L4 males (ncEx9005) were subjected to either control orCeLST8RNAi, and then lysed. FLAG∷LET-363 proteins in the lysate were immunoprecipitated, followed by analysis of IP and lysates. (c) Quantitative ray 1 phenotype in animals overexpressing DAF-15 under thelin-32p in the background ofplx-1orsmp-1 smp-2mutants. (d) Quantitative ray 1 phenotypes caused by loss of LKB1 (par-4), STRAD (strd-1), AMPKα (aak-1&aak-2) or AMPKβ (aakb-1) in the background ofplx-1mutants. (e) Epidermal ray precursor cells visualized withajm-1∷gfpin adaf-15(RNAi) male at the early L4 stage. Anterior is left, and dorsal is top. Scale bar, 10 μm. (f) Nomarski image of a tail in adaf-15(RNAi) adult male. An arrow indicates ray 1; an arrowhead, ray 2. Anterior is left, and dorsal is top. Scale bar, 10 μm. (g) Quantitative ray 1 phenotype in animals subjected to ray-specific RNAi againstplx-1,let-363anddaf-15. Fora,c,d,g: for the quantitative evaluation, the ray 1 phenotypes are categorized into either Level 1 (normal), Level 2 (mildly defective), or Level 3 (severely defective), which are represented by white, grey or black segment of each bar, respectivelyn=148–234 for each genotype. Figure 3: TORC2 inhibition and/or TORC1 activation bypass the SMP signal. ( a ) Quantitative ray 1 phenotype caused by CeLST8 knockdown in the plx-1 mutant background. ( b ) Transgenic L3–L4 males ( ncEx9005 ) were subjected to either control or CeLST8 RNAi, and then lysed. FLAG ∷ LET-363 proteins in the lysate were immunoprecipitated, followed by analysis of IP and lysates. ( c ) Quantitative ray 1 phenotype in animals overexpressing DAF-15 under the lin-32 p in the background of plx-1 or smp-1 smp-2 mutants. ( d ) Quantitative ray 1 phenotypes caused by loss of LKB1 ( par-4 ), STRAD ( strd-1 ), AMPKα ( aak-1 & aak-2 ) or AMPKβ ( aakb-1 ) in the background of plx-1 mutants. ( e ) Epidermal ray precursor cells visualized with ajm-1 ∷ gfp in a daf-15 ( RNAi ) male at the early L4 stage. Anterior is left, and dorsal is top. Scale bar, 10 μm. ( f ) Nomarski image of a tail in a daf-15 ( RNAi ) adult male. An arrow indicates ray 1; an arrowhead, ray 2. Anterior is left, and dorsal is top. Scale bar, 10 μm. ( g ) Quantitative ray 1 phenotype in animals subjected to ray-specific RNAi against plx-1 , let-363 and daf-15 . For a , c , d , g : for the quantitative evaluation, the ray 1 phenotypes are categorized into either Level 1 (normal), Level 2 (mildly defective), or Level 3 (severely defective), which are represented by white, grey or black segment of each bar, respectively n =148–234 for each genotype. Full size image Conversely, we analysed the effects of TORC1 inhibition and TORC2 activation on the ray morphogenesis. Knockdown of TORC1 component genes, let-363 and daf-15 , by a standard RNAi protocol causes developmental arrest [31] , [32] and prevents analysis of the ray morphology. As an alternative strategy, ray-specific RNAi was exploited (Methods). We found that ray-specific RNAi against let-363 and daf-15 caused the ray phenotype to be as penetrant as ray-specific plx-1 RNAi ( Fig. 3e–g ), but did not suppress the plx-1 mutant phenotype ( Supplementary Table S1 ). Likewise, a less pronounced but similar phenotype was observed by the lin-32 p-driven RICT-1 overexpression, which presumably increases TORC2 ( Supplementary Table S1 ). Thus, these results suggest that TORC1 cooperates with SMP signalling whereas TORC2 antagonizes it. Semaphorin shifts the TOR adaptor from Rictor to Raptor Our results led us to speculate that SMP regulates the assembly of the two TORCs. To investigate this possibility, we compared the amount of DAF-15 and that of RICT-1 complexed with LET-363 in lin-32 -expressing ray precursor cells between wild types, plx-1 mutants and smp-1 smp-2 mutants. We retrieved transgenic males at L3–L4 stages, during which ray morphogenesis is controlled by the SMP signal, so as to detect the TORC formation during the SMP-regulated ray morphogenesis. In mutants, the amount of LET-363-bound RICT-1 increased by about 240%, whereas that of LET-363-bound DAF-15 decreased by about 60% of wild types ( Fig. 4a ; Supplementary Fig. S3 ). Restoration of plx-1 expression by heat shock rescued the perturbed TORC formation in plx-1 mutants, whereas it failed to rescue that in smp-1 smp-2 mutants ( Fig. 4a ), probably because of the incapability of PLX-1 alone to transduce the signal in the absence of its ligands. As the total amounts of RICT-1, DAF-15 and LET-363 in the whole lysates were indistinguishable among genotypes ( Fig. 4a ), it is indicated that the SMP signal through PLX-1 serves to promote a shift of the LET-363-associated adaptor from RICT-1 towards DAF-15. By contrast in unc-54 -expressing muscle cells, where PLX-1 expression is absent, significant difference was not observed in the amount of LET-363-bound DAF-15 and RICT-1 between wild types and plx-1 mutants ( Fig. 4b ), confirming the importance of SMP–PLX-1 signalling on TOR partnering. To test further the SMP-regulated TORC formation, we utilized the system of SMP signal reinforcement that can be triggered by simultaneous expression of smp-1 and plx-1 by heat shock, which was previously shown to quickly enhance SMP signalling [7] . Both in ray precursor cells and muscle cells, reinforcement of the SMP signal resulted in a further decrease in LET-363–RICT-1 and an increase in LET-363–DAF-15 association ( Fig. 4c ), indicative of an acute effect of the SMP signal on the TORC formation. 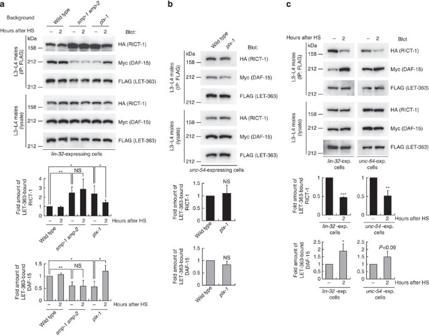Figure 4: The SMP signal promotes a shift of the LET-363-associated adaptor from RICT-1 towards DAF-15. (a) TORC1 and TORC2 formations in wild-type,plx-1andsmp-1 smp-2mutant ray precursor cells. Transgenic L3–L4 males (ncEx9005) in the indicated genetic backgrounds, which carry three TORC component genes under thelin-32p together withplx-1underhsp (hsp∷plx-1), were either untreated (−) or treated with brief heat-shock and collected two hours after heat-shock (2). FLAG∷LET-363 proteins in the lysate were immunoprecipitated, followed by analysis of IP and lysates. The intensity of co-immunoprecipitated HA∷RICT-1 (black bars) or Myc∷DAF-15 (grey bars) normalized by FLAG∷LET-363 in IP is shown in the graphs. Shown are the means±s.e.m. of four independent experiments. (b) TORC1 and TORC2 formations inunc-54-expressing muscle cells in wild-type andplx-1mutants, which were analysed with a line,ncEx9007. The intensity of co-immunoprecipitated HA∷RICT-1 (black bars) or Myc∷DAF-15 (grey bars) normalized by FLAG∷LET-363 in IP is shown in the graphs. Shown in the graphs are the means±s.e.m. of four independent experiments. (c) TORC1 and TORC2 formations under reinforced SMP signalling. The same protocol was employed as ina, except for that the lines carry bothhsp∷smp-1andhsp∷plx-1transgenes.ncEx9011was utilized to analyse the TORC formations inlin-32-expressing cells;ncEx9012, inunc-54-expressing cells. The intensity of co-immunoprecipitated HA∷RICT-1 (black bars) or Myc∷DAF-15 (grey bars) normalized by FLAG∷LET-363 in IP is shown in the graphs. Shown in the graphs are the means±s.e.m. of three independent experiments. One asterisk indicatesP<0.05; two asterisks,P<0.005; three asterisks,P<0.001 for all panels. Pairedt-test was carried out to calculate theP-values. NS, not significant (P>0.05). Figure 4: The SMP signal promotes a shift of the LET-363-associated adaptor from RICT-1 towards DAF-15. ( a ) TORC1 and TORC2 formations in wild-type, plx-1 and smp-1 smp-2 mutant ray precursor cells. Transgenic L3–L4 males ( ncEx9005 ) in the indicated genetic backgrounds, which carry three TORC component genes under the lin-32 p together with plx-1 under hs p ( hs p ∷ plx-1 ), were either untreated (−) or treated with brief heat-shock and collected two hours after heat-shock (2). FLAG ∷ LET-363 proteins in the lysate were immunoprecipitated, followed by analysis of IP and lysates. The intensity of co-immunoprecipitated HA ∷ RICT-1 (black bars) or Myc ∷ DAF-15 (grey bars) normalized by FLAG ∷ LET-363 in IP is shown in the graphs. Shown are the means±s.e.m. of four independent experiments. ( b ) TORC1 and TORC2 formations in unc-54 -expressing muscle cells in wild-type and plx-1 mutants, which were analysed with a line, ncEx9007 . The intensity of co-immunoprecipitated HA ∷ RICT-1 (black bars) or Myc ∷ DAF-15 (grey bars) normalized by FLAG ∷ LET-363 in IP is shown in the graphs. Shown in the graphs are the means±s.e.m. of four independent experiments. ( c ) TORC1 and TORC2 formations under reinforced SMP signalling. The same protocol was employed as in a , except for that the lines carry both hs p ∷ smp-1 and hs p ∷ plx-1 transgenes. ncEx9011 was utilized to analyse the TORC formations in lin-32 -expressing cells; ncEx9012 , in unc-54 -expressing cells. The intensity of co-immunoprecipitated HA ∷ RICT-1 (black bars) or Myc ∷ DAF-15 (grey bars) normalized by FLAG ∷ LET-363 in IP is shown in the graphs. Shown in the graphs are the means±s.e.m. of three independent experiments. One asterisk indicates P <0.05; two asterisks, P <0.005; three asterisks, P <0.001 for all panels. Paired t -test was carried out to calculate the P -values. NS, not significant ( P >0.05). Full size image To test whether decreased TORC1 and increased TORC2 in plx-1 mutant ray precursor cells are associated with changes in their activities, we monitored a phosphorylation state of a TORC1 substrate, 4EBP [19] , and that of a TORC2 substrate, PKCα [13] , [23] . As SPN-2, a putative counterpart of the translational repressor 4EBP1 (ref. 37 ), and four PKC proteins encoded by pkc-1 (PKCɛ), pkc-2 (PKCα), pkc-3 (PKCι) and tpa-1 (PKCδ) [38] , cannot be recognized by commercially available antibodies, an alternative strategy to monitor the C. elegans TORC activities was adopted by utilizing a line expressing human 4EBP1 (h4EBP1) or rat PKCα (rPKCα) tagged with FLAG and placed under the lin-32 p. These xenogeneic molecules appeared to serve as substrates for C. elegans TORCs, because let-363 and daf-15 knockdowns abolished h4EBP1 phosphorylation (P-h4EBP1) whereas let-363 knockdown and rict-1 mutation abolished P-rPKCα ( Fig. 5a ). In plx-1 mutants, P-h4EBP1 reduced by about 60%, whereas P-rPKCα increased by about 150% of wild types ( Fig. 5a ), which seemingly correlates with decreased TORC1 and increased TORC2 formations in mutants. Taken together, these results indicate that SMP signalling activates TORC1 whereas it inactivates TORC2 by shifting the LET-363-associated adaptor from RICT-1 to DAF-15. 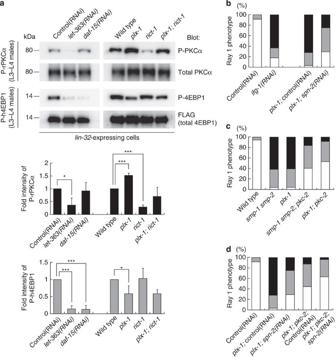Figure 5: SMP signalling necessitates both TORC1 activation and TORC2 inactivation. (a) Phosphorylation of xenogeneically expressed rat PKCα (rPKCα) and human 4EBP1 (h4EBP1) inlin-32-expressing cells were used to assess the activities of TORC2 and TORC1, respectively. L3–L4 males in the indicated genetic background carrying either thelin-32p∷FLAG∷rPKCα transgene (ncEx9014) or thelin-32p∷FLAG∷h4EBP1transgene (ncEx9013) were lysed, and analysed for their phosphorylation states by immunoblotting. Black bars represent normalized P-rPKCα; grey bars, normalized P-h4EBP1. Shown in the graphs are the means±s.e.m. of three independent experiments. One asterisk indicatesP<0.05; three asterisks,P<0.001. Pairedt-test was carried out to calculate theP-values. (b) Quantitative ray 1 phenotypes in wild-type adults subjected toifg-1RNAi andplx-1mutant adults subjected tospn-2RNAi. (c) Quantitative ray 1 phenotypes caused by loss ofpkc-2function in the genetic background ofplx-1orsmp-1 smp-2mutants. (d) Quantitative ray 1 phenotypes ofspn-2andpkc-2double knockdown in the genetic background ofplx-1mutants. Forb–d: for the quantitative evaluation, the ray 1 phenotypes are categorized into either Level 1 (normal), Level 2 (mildly defective), or Level 3 (severely defective), which are represented by white, grey or black segment of each bar, respectively.n=105–234 for each genotype. Figure 5: SMP signalling necessitates both TORC1 activation and TORC2 inactivation. ( a ) Phosphorylation of xenogeneically expressed rat PKCα (rPKCα) and human 4EBP1 (h4EBP1) in lin-32 -expressing cells were used to assess the activities of TORC2 and TORC1, respectively. L3–L4 males in the indicated genetic background carrying either the lin-32 p ∷ FLAG ∷ rPKC α transgene ( ncEx9014 ) or the lin-32 p ∷ FLAG ∷ h4EBP1 transgene ( ncEx9013 ) were lysed, and analysed for their phosphorylation states by immunoblotting. Black bars represent normalized P-rPKCα; grey bars, normalized P-h4EBP1. Shown in the graphs are the means±s.e.m. of three independent experiments. One asterisk indicates P <0.05; three asterisks, P <0.001. Paired t -test was carried out to calculate the P -values. ( b ) Quantitative ray 1 phenotypes in wild-type adults subjected to ifg-1 RNAi and plx-1 mutant adults subjected to spn-2 RNAi. ( c ) Quantitative ray 1 phenotypes caused by loss of pkc-2 function in the genetic background of plx-1 or smp-1 smp-2 mutants. ( d ) Quantitative ray 1 phenotypes of spn-2 and pkc-2 double knockdown in the genetic background of plx-1 mutants. For b – d : for the quantitative evaluation, the ray 1 phenotypes are categorized into either Level 1 (normal), Level 2 (mildly defective), or Level 3 (severely defective), which are represented by white, grey or black segment of each bar, respectively. n =105–234 for each genotype. Full size image Semaphorin signalling through active TORC1 and inactive TORC2 Previously, we showed that knockdown of ifg-1 (eIF4G; a component of eIF4F complex) phenocopies plx-1 and smp-1 smp-2 mutants, whereas knockdown of spn-2 (4EBP; a translational repressor) partially suppresses the plx-1 mutant phenotype ( Fig. 5b ) [7] . Taking these findings together with our present result of reduced P-h4EBP1 in plx-1 mutants, we reasoned that increased and thus upregulated TORC1 mediates the SMP signal by repressing SPN-2 and activating translation. However, loss of S6K ( rsks-1 ), another putative TORC1 substrate [19] , did not cause ray defects ( Supplementary Fig. S4a ). This result rules out possible contribution of S6K to SMP signalling, and is consistent with a previous report arguing against C. elegans S6K as the TOR downstream mediator [31] . Next, to investigate the biological relevance of SMP-induced TORC2 downregulation, we disrupted PKC, a putative TORC2 substrate [13] , [23] . Striking but not full suppression of the plx-1 and smp-1 smp-2 mutant phenotype was observed by pkc-2 and pkc-3 deficiency ( Fig. 5c ; Supplementary Fig. S4b ). Loss of the other PKC isoforms, pkc-1 and tpa-1 , did not significantly affect the smp-1 smp-2 mutant phenotype ( Supplementary Fig. S4b ). Thus, inhibition of PKCα and possibly PKCι caused by TORC2 downregulation is suggested to be another means by which SMP signalling controls the proper ray morphogenesis. Intriguingly, simultaneous inhibition of spn-2 and pkc-2 suppressed the plx-1 mutant phenotype more strikingly than either single inhibition ( Fig. 5d ), supporting an idea that SMP signalling requires both TORC1 activation and TORC2 inactivation. We also analysed roles of AKTs ( akt-1 & akt-2 ) [39] , well-defined TORC2 substrates [21] , and FoxO ( daf-16 ), a putative AKT effector [39] , on SMP-mediated ray positioning. Unexpectedly, their deficiencies neither caused the ray 1 phenotype nor suppressed the plx-1 mutant phenotype ( Supplementary Fig. S4c ), excluding the idea that AKT-FoxO signalling is involved in the SMP–TORC2 pathway. As previously suggested [30] , AKTs may not be the primary effectors of TORC2 in C. elegans . Finally, we examined whether the activity of eIF2, another translation factor that participates in translation initiation and has been shown to mediate the SMP signal [7] , is also under the control of TORCs. We observed higher phosphorylation of its α subunit (eIF2α), representing diminished global translation, in let-363 and daf-15 knockdowns similar to plx-1 mutants ( Fig. 6 ). Thus, through an as yet unknown mechanism, TORC1 seems to serve as a central mediator of SMP-stimulated mRNA translation through eIF2. 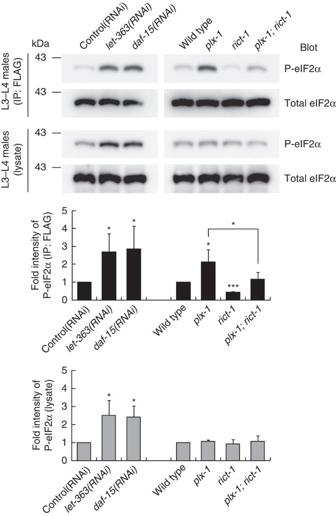Figure 6: eIF2α phosphorylation is influenced by the TOR complex signal. L3–L4 males carrying thelin-32p∷eIF2α∷FLAGtransgene (ncEx9002) were lysed, and FLAG-tagged eIF2α proteins were immunoprecipitated and subjected to immunoblot analysis with antibodies against total eIF2α or phospho-eIF2α. Black bars represent P-eIF2α in IP; grey bars, in lysate. Shown in the graphs are the means of normalized P-eIF2α±s.e.m. of three independent experiments. One asterisk indicatesP<0.05; three asterisks,P<0.001. Pairedt-test was carried out to calculate theP-values. Figure 6: eIF2α phosphorylation is influenced by the TOR complex signal. L3–L4 males carrying the lin-32 p ∷ eIF2 α ∷ FLAG transgene ( ncEx9002 ) were lysed, and FLAG-tagged eIF2α proteins were immunoprecipitated and subjected to immunoblot analysis with antibodies against total eIF2α or phospho-eIF2α. Black bars represent P-eIF2α in IP; grey bars, in lysate. Shown in the graphs are the means of normalized P-eIF2α±s.e.m. of three independent experiments. One asterisk indicates P <0.05; three asterisks, P <0.001. Paired t -test was carried out to calculate the P -values. Full size image By contrast to extensive understandings on regulation of TORC1, that of TORC2 has remained poorly characterized. Here we provide the genetic demonstration of an aspect of TORC2 regulation in C. elegans . We showed that TORC2 is downregulated by the morphogenetic semaphorin signal, and this coincides with TORC1 upregulation, which are based on semaphorin-induced concerted alteration in biochemical assemblies of the two TORCs. Our present study began with isolation of Rictor deficiency as a suppressor of the plexin mutant ray phenotype, providing us with a clue to the semaphorin action on TOR. Akin to Rictor deficiency, Raptor overexpression suppressed the semaphorin and plexin mutant phenotype. Conversely, animals deficient in Raptor and TOR, as well as animals overexpressing Rictor, were phenotypically similar to semaphorin and plexin mutants, indicating that TORC1 cooperates with whereas TORC2 antagonizes semaphorin signalling. A key finding is that Raptor–TOR association was diminished whereas Rictor–TOR association was facilitated in semaphorin and plexin mutants, along with TORC1 down- and TORC2 up-regulation. Moreover, reinforcement of semaphorin input in the wild-type background was sufficient to quickly diminish TORC2 while facilitating TORC1 assembly. Since the total amounts of Rictor and Raptor were indistinguishable, irrespective of semaphorin input, our results indicate that semaphorin post-translationally shifts the TOR adaptor from Rictor towards Raptor ( Fig. 7 ). 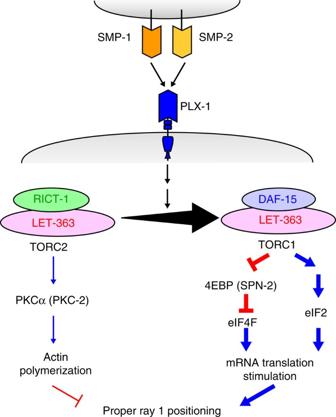Figure 7: A model illustrating semaphorin signalling through TOR leading to morphogenetic changes in epidermal cells. The semaphorin signal through plexin promotes a shift of the LET-363 adaptor from RICT-1 towards DAF-15. Increase in the level of TORC1 culminates in translation stimulation of mRNAs. This involves activation of eIF4F by inhibiting its negative regulator 4EBP through phosphorylation, as well as activation of eIF2 by reducing phosphorylation of eIF2α. Concomitantly, decrease in the level of TORC2 reduces the level of phospho-PKCα, which probably leads to destabilization of actin cytoskeleton. Figure 7: A model illustrating semaphorin signalling through TOR leading to morphogenetic changes in epidermal cells. The semaphorin signal through plexin promotes a shift of the LET-363 adaptor from RICT-1 towards DAF-15. Increase in the level of TORC1 culminates in translation stimulation of mRNAs. This involves activation of eIF4F by inhibiting its negative regulator 4EBP through phosphorylation, as well as activation of eIF2 by reducing phosphorylation of eIF2α. Concomitantly, decrease in the level of TORC2 reduces the level of phospho-PKCα, which probably leads to destabilization of actin cytoskeleton. Full size image What are the molecular consequences of alteration in the ratio of TORC1 to TORC2 by semaphorin? Activated TORC1 augments translation by phosphorylating and antagonizing a translation inhibitor 4EBP [19] . We observed decreased P-h4EBP1 in plexin mutants, which appeared relevant to decreased TORC1. In addition, 4EBP knockdown suppressed the ray defect in plexin mutants. Thus, we propose that semaphorin stimulates translation through TORC1-mediated negative regulation on 4EBP. This is consistent with our previous finding of a role for semaphorin in translation stimulation through another translation factor, eIF2α [7] . Moreover, compelling evidence came from studies on vertebrate neurons, which showed that semaphorin triggers 4EBP phosphorylation and stimulates translation [5] , [6] . A TORC1 inhibitor rapamycin blocks the semaphorin-induced growth cone responses [5] , in agreement with our finding that Raptor and TOR deficients phenocopied semaphorin and plexin mutants. Another intriguing observation is that TORC1 inhibition (TOR and Raptor knockdowns) not only decreased P-h4EBP1 but elevated P-eIF2α, implicating a cross-talk between the two regulatory pathways for translation by TORC1. This is reminiscent of reports that rapamycin inhibits TAP42 phosphatase complex-associated TORC1, resulting in translation repression through increased eIF2α phosphorylation [40] , [41] . Therefore, we postulate that the semaphorin signal is integrated and diverged by TORC1 into activation of eIF2 and eIF4F systems, which subsequently converges to promote translation. Growing evidence suggests that TORC2 modulates cytoskeleton-based events, including cell morphogenesis and migration [13] , [14] , [20] , [42] , [43] . These events are mediated in part by Rho GTPases and PKC, which eventually induce actin polymerization. Here we report PKCα/PKC-2 and PKCι/PKC-3 as candidate substrates for TORC2, whose activities are diminished by semaphorin input. Thus, we consider that the semaphorin signal is conveyed into destabilization of actin architecture through inhibition of the TORC2–PKC pathway. In agreement with this, we and others demonstrated that activation–inactivation cycling and de novo synthesis of cofilin, an actin-depolymerizing factor, underlie the semaphorin-induced morphological events [7] , [8] , [44] . In motile Dictyostelium , TORC2 regulation is confined to the leading edges of cAMP-oriented cells, where cytoskeleton-related proteins are dynamically regulated by TORC2 (refs 42 , 45 ). It is interesting to speculate that semaphorin-induced inhibition of the TORC2–PKC pathway attenuates the rate of F-actin formation at the R1.p–R2.p boundary. Concertedly, semaphorin increases TORC1 and thereby translationally activates cytoskeleton-relevant proteins like cofilin, which enables acceleration of actin depolymerization locally at the cell–cell contact sites and allows for the proper positioning of ray 1. As our results and a previous report illustrate [46] , the choice of TOR partners between Raptor and Rictor seems to be controlled by physiological stimuli, serving as an important step in the regulation of the two TORCs signalling pathways. The precise molecular mechanism by which TORC assembly is regulated remains to be elucidated at present. We found that Raptor and Rictor are in a competitive relationship for binding to TOR, though the results obtained with overexpressing transgenes might not strictly reflect physiological conditions. This may imply that semaphorin mediates conversion of TORC2 to TORC1 simply by either destabilizing TORC2 or stabilizing TORC1 through biochemical modulation of the TORC components. In mammalian cells, competitive binding is implicated, at least partly, in FoxO-mediated regulation of assembly of mTOR complexes [46] . Otherwise, localization of the TORC components might be the basis for semaphorin-induced shift of the TOR adaptors. Recently, several reports have demonstrated the importance of changes in the subcellular localization of two TORCs on their functionalities. Rag GTPase-bound TORC1 is recruited from dispersed puncta to endomembrane structure on nutritional stimuli, where it is activated by Rheb [47] . In endothelial cells, Syndecan-4, a membrane-bound proteoglycan, targets TORC2 to membrane rafts, thereby rendering TORC2 active but TORC1 inactive [48] . It might be possible that semaphorin delocalizes and thus inactivates TORC2 while relocalizing TORC1 to its active sites. In the future, analysis of the subcellular localization of TOR and/or the TOR adaptors within ray precursor cells may provide more clues to the mechanism of the semaphorin action on TOR. In conclusion, we have demonstrated genetic and biochemical evidence of TOR partnering by semaphoring–plexin signalling during cellular morphogenesis in C. elegans . Semaphorin-activated TORC1 augments translation through eIF4F as well as eIF2 activation, and concomitant TORC2 inhibition probably results in F-actin destabilization ( Fig. 7 ). Therefore, we propose that TOR has a central role in integrating upstream semaphorin input and subsequently transducing the signal into divergent multiple downstream cascades. Strains C. elegans culture and genetics were performed as described by Brenner [49] . To facilitate the analyses of males, all strains carried him-5 ( e1490 ) or him-8 ( e1489 ). The following alleles were used in this study: [LGI] smp-1 ( ev715 ), smp-2 ( ev709 ), daf-16 ( mu86 ); [LGII] rict-1 ( nc41 ), rrf-3 ( pk1426 ), ncIs13 [ ajm-1 ∷ gfp ]; [LGIII] aak-1 ( tm1944 ), strd-1 ( ok2283 ), rsks-1 ( tm1714 ); [LGIV] plx-1 ( nc37 ), tpa-1 ( k529 ), him-8 ( e1489 ); [LGV] pkc-1 ( nj1 ), rde-1 ( km56 ), par-4 ( it57 ), him-5 ( e1490 ); [LGX] pkc-2 ( ok328 ), aak-2 ( ok524 ), aakb-1 ( tm2658 ), ncIs35 [ lin-32 p ∷ rde-1 ∷ egfp ]; Bristol N2 and Hawaiian CB4856. Isolation and characterization of rict-1 ( nc41 ) mutants Suppressor screening was performed through mutagenesis on plx-1 ( nc37 ); him-5 ( e1490 ) mutants with ethyl methanesulfonate [7] . One isolated suppressor, nc41 , was out-crossed more than ten times. nc41 single mutants were fertile and appeared healthy, but the brood size was reduced to 60% of wild-type N2 (N2: 275.8±25 ( n =4); nc41 : 161.7±25 ( n =12)). Two-factor and three-factor crosses mapped nc41 at about 8 map units right to rol-1 and about 9 map units left to unc-52 on linkage group II. Further mapping was performed by utilizing SNPs between N2 and CB4856 strains. Using genomic DNA from 169 populations, nc41 was mapped between nucleotide (nt:) 12,398 on Y81G3A and nt: 18,109 on F32A11 (about 56 kbp). PCR using genomic DNA from nc41 mutant populations as template failed to amplify DNA fragments around nt: 2,969 on F29C12, indicating that this region was deleted in nc41 . Subsequent sequencing revealed that nc41 was a deletion between nt: 13,469 and nt: 13,938 (470 bp) within F29C12.3 gene ( rict-1 ). RNA interference A cDNA fragment of plx-1 (nt: 603–1,912), rict-1 (nt: 1–892), daf-15 (nt: 1–555), let-363 (nt: 1–536), CeLST8 /C10H11.8 (nt: 9–1,130), pkc-3 (nt: 10–1,780), akt-1 (nt: 5–747), akt-2 (nt: 18–1,387), spn-2 (nt: 29–1,077), or a genomic DNA fragment of ifg-1 (M110: 15,908–16,949) was subcloned into the pPD129.36 vector, and the resultant plasmids were transformed into the HT115 bacterial strain [50] . L4 hermaphrodites were grown on lawns of the transformed bacteria, and the F1 progeny were analysed for their phenotypes. Culture plates seeded with bacteria harbouring the empty pPD129.36 vector were used as controls. For the microscopic observation of rays, RNAi was performed in the background of rrf-3 ( pk1426 ), which gives hypersensitivity to RNAi [51] . For the ray-specific RNAi experiments, we used a line rrf-3 ( pk1426 ); rde-1 ( km56 ); ncIs35 [ lin-32 p ∷ rde-1 ∷ egfp ], where the RNAi-defective phenotype caused by rde-1 mutation is rescued specifically in lin-32 -expressing ray precursor cells [52] . Immunoprecipitation L3 and L4 males were collected in IP lysis buffer containing 40 mM HEPES (pH7.5), 120 mM NaCl, 1 mM EDTA and 0.3% CHAPS supplemented with 1 mM PMSF and protease inhibitor cocktail (Sigma), and dissolved by sonication (5-s sonication with a 5-s break, 10 cycles) and incubation with constant rotation for two hours at 4 °C. FLAG-tagged proteins were immunoprecipitated with anti-FLAG M2 affinity gel (Sigma) as per the manufacturer's instruction. To immunoprecipitate Myc- or HA-tagged proteins, lysates were precleared with protein G-agarose (Roche Applied Science) for two hours at 4 °C, and incubated with anti-Myc (9E10) or anti-HA (Roche Applied Science) antibodies overnight at 4 °C. Samples were then incubated again with protein G-agarose for another two hours at 4 °C, to allow for the precipitation. Immunoprecipitates were washed with CHAPS-free IP lysis buffer three times at 4 °C, and then eluted by boiling with 2× SDS sample buffer at 95 °C for 3 min. Both immunoprecipitates and lysates were subjected to subsequent western blot analysis. Western blot analysis Samples were run on 6 or 9% SDS–PAGE and transferred to an Immobilon-P PVDF membrane (Millipore). Western blots were probed overnight at 4 °C with rabbit anti-FLAG (Sigma), mouse anti-Myc (9E10), mouse anti-HA (Roche), rabbit anti-phospho-4EBP1 (Cell Signaling Technology), rabbit anti-PKCα (Santa Cruz), rabbit anti-phospho-PKCα (Upstate), rabbit anti-eIF2α [7] , or rabbit anti-phospho-eIF2α (Cell Signaling) primary antibodies. The blots were visualized by incubation for two hours at room temperature with HRP-conjugated anti-mouse or anti-rabbit IgG secondary antibodies (Cell Signaling), followed by detection with an Immobilon Western chemiluminescent HRP substrate (Millipore). Images were captured and quantified with Luminescent Image Analyser LAS-4000 (Fujifilm). Paired t -test was used to evaluate differences in the signal intensities. Heat-shock-induced gene expression L3 and L4 males carrying the extrachromosomal hs p ∷ plx-1 and/or hs p ∷ smp-1 transgenes on NGM plates were heat-shocked for 15 min at 37 °C. Animals were collected two hours after heat-shock and subjected to Western blot analysis. cDNA construction Full-length wild-type rict-1 cDNA was constructed by fusing the 5′ RACE product corresponding to the 1st–12th exons with the 3′ cDNA yk1311f01 covering the ninth exon through 3′UTR of the gene, which was kindly provided by Yuji Kohara. To clone nc41 -type rict-1 cDNA, we extracted poly(A) RNAs from nc41 mutants, reverse-transcribed the mRNAs using oligo-d(T) primer, and identified opal codon at the position 1,200th in the mutant rict-1 cDNA. Then, 3′ moiety of the mutant cDNA was PCR-amplified and digested with Bsp EI/ Eco RV enzymes, with which the equivalent region of the wild-type rict-1 cDNA was replaced. Full-length wild-type daf-15 cDNA was constructed by fusing the 5′ RACE product corresponding to the 1st–5th exons with yk1462 covering the 3rd–12th exons and yk893 covering the eighth exon through 3′UTR of the gene. Full-length wild-type let-363 cDNA was constructed by fusing the 5′ RACE product with the 3′ cDNA yk22f1 . These cDNAs were modified to be flanked by Kpn I sites at both ends to facilitate the subsequent subcloning. Primer sequences for the generation of these cDNAs are available on request. Generation of transgenic lines The pPD49.78 and the pPD30.38 vectors were used to express genes of interest under the heat-shock promoter ( hs p 16-2 ) and the unc-54 promoter, respectively. The lin-32 promoter-inserted pPD49.26 vector was used to express genes in ray precursor cells [7] , [28] . FLAG , Myc , or HA adaptor sequence was fused to the 5′ end of cDNAs. The epitope-tagged daf-15 and rict-1 genes placed under the lin-32 p are suggested to be functional, because they exerted the same effects on ray morphogenesis as their corresponding untagged ones ( Supplementary Table S1 ). Each of the following DNAs flanked by synthetic restriction sites was inserted into the multiple cloning sites of each vector. The transgene harbouring cDNA for plx-1 , smp-1 , rict-1 (with or without a HA tag), daf-15 (with or without a Myc tag), let-363 (FLAG-tagged), human 4EBP1 (FLAG-tagged), or rat PKCα (FLAG-tagged) was mixed with pRF4 and injected into gonads of N2 hermaphrodites to establish stable extrachromosomal arrays [53] . The lin-32 p ∷ rde-1 ∷ egfp transgene was injected together with pRF4 to establish an extrachromosomal array, which was then chromosomally integrated by γ -ray irradiation [54] to generate ncIs35 . Extrachromosomal arrays used and the final concentrations of the transgenes for injection are listed on Supplementary Table S2 . Primer sequences for the generation of the transgenes are available on request. Microscopy Animals were mounted on 4% agar pads containing 1 mM levamisole for immobilization. Ray phenotypes at the adult stage were analysed with Nomarski differential interference optics (ZEISS Axioplan 2). Images were captured with a Penguin 600CL CCD camera (Pixera). GFP expressions at the cell boundaries of epidermal ray precursor cells in ncIs13 were scored and captured with a confocal microscopy Olympus Fluoview300. Phenotypic analysis of ray 1 Three 'levels' (Level 1, Level 2, Level 3) were used as criteria for the quantitative evaluation of the ray 1 phenotype [7] . Briefly, level 1 refers to a normal state where ray 1 is closely situated to its neighbouring ray 2. Level 2 refers to a mildly defective state where ray 1 is separated from ray 2 within a cuticular fan. Level 3 refers to a severely defective state where ray 1 is situated apart from ray 2 outside of a fan. Fisher's exact test was used to statistically evaluate differences in the ray 1 phenotype between two genotypes ( Supplementary Table S1 ). How to cite this article: Nukazuka, A. et al . A shift of the TOR adaptor from Rictor towards Raptor by semaphorin in C. elegans . Nat. Commun. 2:484 doi: 10.1038/ncomms1495 (2011).